A polysaccharide bioprotonic field-effect transistor In nature, electrical signalling occurs with ions and protons, rather than electrons. Artificial devices that can control and monitor ionic and protonic currents are thus an ideal means for interfacing with biological systems. Here we report the first demonstration of a biopolymer protonic field-effect transistor with proton-transparent PdH x contacts. In maleic-chitosan nanofibres, the flow of protonic current is turned on or off by an electrostatic potential applied to a gate electrode. The protons move along the hydrated maleic–chitosan hydrogen-bond network with a mobility of ~4.9×10 −3 cm 2 V −1 s −1 . This study introduces a new class of biocompatible solid-state devices, which can control and monitor the flow of protonic current. This represents a step towards bionanoprotonics. Proton (H + ) transport is important in many natural phenomena [1] . Preeminent examples include ATP oxidative phosphorylation in mithochondria [2] , the HCVN1 voltage-gated proton channel [3] , light-activated proton pumping in bacteriorhodopsin [4] , and the proton-conducting single water file in the antibiotic gramicidin [5] . In living systems, electrical signals are communicated and processed by modulating ionic [6] and protonic currents [7] . In contrast, the development of computing has mainly focused on devices that control electronic currents such as vacuum tubes, solid-state field-effect transistors (FET), and nanoscale molecular structures [8] , [9] , [10] , [11] . Few examples of protonic-based devices exist, and include an ice FET working with AC current [12] , and a water bipolar junction transistor [13] . At the nanoscale, ionic (and protonic) conductivity has attracted increasing interest with the advent of resistive ionic memories [14] , memristors [15] , [16] , synaptic transistors [17] , and nanofluidics [18] , [19] , [20] . In hybrid bionanodevices, biological multifunctionality has been added to carbon nanotubes [21] or silicon nanowires [22] with transmembrane proton conductive proteins. Bionanoelectronic devices [23] that can control the current of ions and protons—a more appropriate language than electrons in nature [24] —are uniquely positioned. In this regard, nanofluidics devices are particularly attractive. However, these require microscopic liquid reservoirs, and current control at physiological concentration is limited to difficult-to-fabricate nanometer channels [20] . Recently, conducting polymer ion bipolar junction transistor devices have been demonstrated [25] , [26] . These exploit ion selective membranes as contacts to extract and deliver ions (Na + , K, + Ca 2+ ) and neurotransmitters in solution. To further this exciting route, biocompatible field-effect devices with H + -selective solid-state contacts would allow exclusive interfacing with biological proton-conducting channels. Here we demonstrate a new class of solid-state H + -FET devices that afford electrostatic control of the protonic current ( Fig. 1 ). In our maleic–chitosan H + -FET, the flow of protonic current—measured with proton transparent palladium hydride (PdH x ) (ref. 27 ) contacts—is turned on or off by an electrostatic potential applied to the gate electrode. Protons dissociated from the maleic acid groups move along the hydrated molecule hydrogen-bond network following the Grotthus mechanism [2] (mobility, μ H+ ≈4.9×10 −3 cm 2 V −1 s −1 ). 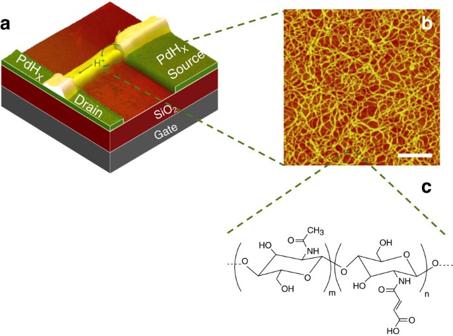Figure 1: Schematics and atomic force micrographs of protonic field-effect transistors. (a) AFM image (false coloured) overlayed onto a schematic of bottom contact back-gated transistor type device. PdHxcontacts (10 μm wide, 8.6 μm spacing) are on the top of a 100 nm SiO2capping a p-type (0.001 ohm cm−1) wafer. maleic–chitosan thin-film dimensions 3.5 μm wide, 8.6 μm long, and 82 nm thick. (b) Atomic force micrograph of maleic–chitosan nanofibres after partial dissolution of the polysaccharide in water (scale bar 200 nm). (c) Molecular structure of maleic–chitosan, the degree of substitution (m/n) is 0.85 for these devices. Figure 1: Schematics and atomic force micrographs of protonic field-effect transistors. ( a ) AFM image (false coloured) overlayed onto a schematic of bottom contact back-gated transistor type device. PdH x contacts (10 μm wide, 8.6 μm spacing) are on the top of a 100 nm SiO 2 capping a p-type (0.001 ohm cm −1 ) wafer. maleic–chitosan thin-film dimensions 3.5 μm wide, 8.6 μm long, and 82 nm thick. ( b ) Atomic force micrograph of maleic–chitosan nanofibres after partial dissolution of the polysaccharide in water (scale bar 200 nm). ( c ) Molecular structure of maleic–chitosan, the degree of substitution ( m /n) is 0.85 for these devices. Full size image Device architecture These H + -FET devices comprise a maleic–chitosan nanofibre protonic channel bridging PdH x contacts (source and drain) on the top of SiO 2 (gate dielectric). Maleic–chitosan (poly (β-(1,4)-N-Maleoyl- D -glucosamine)) ( Fig. 1b,c ) is a polysaccharide chitin derivative of particular interest for the prospect of bionanoprotonics. Most chitin derivatives are biodegradable, nontoxic, and physiologically inert [28] . Palladium is chosen as the contact material for its ability to form proton-conducting PdH x on exposure to hydrogen [27] . PdH x affords proton exchange between the contacts and the maleic–chitosan channel without electrolysis. The SiO 2 (100-nm) gate dielectric insulates the maleic–chitosan and the contacts from the Si electrostatic back gate. Two-terminal measurements We first probe the maleic–chitosan conductivity in thicker films sandwiched by PdH x contacts, to verify that this H + -FET architecture indeed measures protonic current. When a bias is applied between the contacts, the current increases with relative humidity (and polysaccharide hydration level) ( Fig. 2a ). Hysteresis also increases with humidity, potentially due to increased charge accumulation/depletion at the contacts. Measurements using hydrogen-depleted Pd or Au contacts—both proton blocking—record a considerably smaller current ( Supplementary Fig. S1 ). It is important to note that both Au and Pd are significantly better electronic conductors than PdH x . We thus confirm that PdH x contacts effectively measure the protonic current in this material. Increase in protonic conductivity with hydration level is common in other biological macromolecules such as collagen [29] , cellulose [30] and keratin [31] . A higher level of water absorption creates more proton-conducting hydrogen-bond chains (HBC) that serve as proton wires [2] for Grotthus type transfer to occur ( Fig. 2b ). In maleic–chitosan, we propose that the protons responsible for the current (as hydronium ions in the HBC) originate from the polysaccharide maleic acid groups, some of which are deprotonated ( Fig. 2c ). The protonic conductivity in chitin ( Supplementary Fig. S1 ), which has no maleic groups, is significantly lower than in the maleic–chitosan derivative. 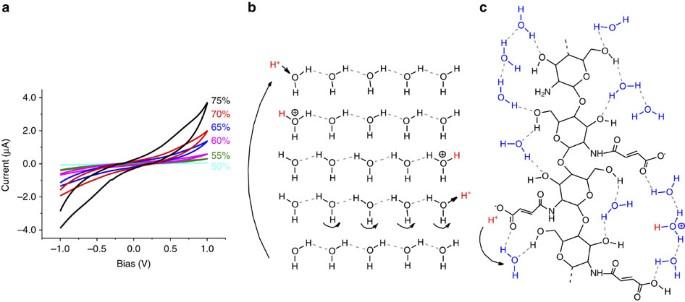Figure 2: Proton conductivity and mechanism. (a) Conductivity as a function of humidity for a maleic–chitosan thin film (1 cm2×1 cm2, 300 μm thick) sandwiched between PdHxelectrodes. (b) Grotthuss mechanism for H+conduction along the hydrogen bonds formed by water and polysaccharide polar groups. (c) A four-monomer segment of maleic–chitosan. The intra- and inter-molecular hydrogen bonds as well as the hydrogen bonds between the water of hydration and the polar parts of the molecule form a continuous network comprised by hydrogen-bond chains. The maleic group donates a H+to the hydrogen-bond network and forms an H3O+(hydronium) ion. Figure 2: Proton conductivity and mechanism. ( a ) Conductivity as a function of humidity for a maleic–chitosan thin film (1 cm 2 ×1 cm 2 , 300 μm thick) sandwiched between PdH x electrodes. ( b ) Grotthuss mechanism for H + conduction along the hydrogen bonds formed by water and polysaccharide polar groups. ( c ) A four-monomer segment of maleic–chitosan. The intra- and inter-molecular hydrogen bonds as well as the hydrogen bonds between the water of hydration and the polar parts of the molecule form a continuous network comprised by hydrogen-bond chains. The maleic group donates a H + to the hydrogen-bond network and forms an H 3 O + (hydronium) ion. Full size image H + -FET measurements In a H + -FET type device, the source-drain protonic current, I ds , recorded as a function of drain-source bias, V ds , is modulated by changing the potential of the back gate electrode, V gs ( Fig. 3 ). As expected for a semiconducting FET with predominantly positive charge carriers, a negative V gs results in a higher source-drain current for the same V ds , whereas a positive V gs almost turns I ds off. In most materials, protons have to overcome activation energy in the range of 0.1 to 1 eV for current to flow [29] , [31] , [32] . This activation energy may be associated with producing a H + OH +− pair or with transport of H + along the HBC. This behaviour is often referred to as protonic semi-conductivity. However, in highly conducting proton wires, such as in gramicidin, the activation energy associated with transport is very small [5] . In the maleic–chitosan pro-FET, the linear I ds dependence on V ds for low V ds (and V gs =0 V) indicates that protons do not need to overcome any appreciable energy barrier for I ds to flow ( Fig. 3a ). This suggests that highly efficient proton wires are formed in the material. 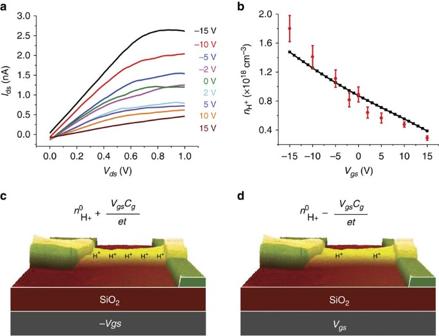Figure 3: Protonic transistors transfer characteristics. (a) Plot ofIdsas a function ofVdsfor differentVgs(RH 75%). For device with PdHxcontacts shown inFigure 1. (b) Plot of channel proton density (nH+) as function of Vgs. Points arenH+derived fromIds–Vdsdata (a) assuming a mobility of (4.9±0.5)×10−3cm2V−1s−1fromn0H+=8.9×1017cm−3atVgs=0. Line is(Cg=gate capacitance per unit area,t=device thickness). From simulationsCg×area=1.79×10−14F. (c,d) Schematics of protonic transistor channel charge carriernH+modulation for negative (c) and positive (d) gate voltage. Figure 3: Protonic transistors transfer characteristics. ( a ) Plot of I ds as a function of V ds for different V gs (RH 75%). For device with PdH x contacts shown in Figure 1 . ( b ) Plot of channel proton density ( n H+ ) as function of V gs . Points are n H+ derived from I ds –V ds data ( a ) assuming a mobility of (4.9±0.5)×10 −3 cm 2 V −1 s −1 from n 0 H+ =8.9×10 17 cm −3 at V gs =0. Line is ( C g =gate capacitance per unit area, t =device thickness). From simulations C g ×area=1.79×10 −14 F. ( c , d ) Schematics of protonic transistor channel charge carrier n H+ modulation for negative ( c ) and positive ( d ) gate voltage. Full size image H + -FET model A simple model can be used to describe the H + -FET. I ds is proportional to V ds through the conductivity of the channel σ = e n H+ μ H+ ( e =proton charge, n H+ =number of free protons per unit volume, and μ H+ =proton mobility). For V gs =0 V, we assume that all the protons available for conduction originate from the maleic acid groups in the polysaccharide (pKa=3.2) ( Supplementary Methods ). From this assumption, we estimate . Using , the proton mobility can be calculated from the slope of I ds at V gs =0 V ( Supplementary Methods ). The calculated value μ H+ ≈4.9×10 −3 cm 2 V −1 s −1 is consistent with the mobility of H + in diluted acidic solutions. [33] For a negative V gs , a positive charge is induced onto the channel because the maleic–chitosan and the gate create a capacitor with the SiO 2 as the dielectric. The charge per unit area induced onto the channel is directly proportional to V gs through the gate capacitance per unit area, C g . To create that charge, excess protons are injected into the maleic–chitosan via the proton transparent contacts. The contribution of these excess protons to the conductivity can then be estimated as an increase in n H+ (higher I ds ) by a factor that is equal to −( V gs C g / et ) ( t =device thickness) ( Fig. 3c ). At the same time, a decrease in n H+ (smaller I ds ) is expected for a positive V gs ( Fig. 3d ). The data in Figure 3b corroborates this description. This plot depicts n H+ estimated from the I ds –V ds experimental data ( Fig. 3a ) as a function of V gs . These n H+ values are compared with , which is the contribution to n H+ expected from the excess charge induced onto the channel by V gs . Given that this model involves several assumptions and approximate estimates of the maleic–chitosan channel volume, this data is in good, even fortuitous, agreement. Measurements performed on a thicker device show a significantly smaller I ds modulation from V gs , as predicted by our description ( Supplementary Fig. S2 ). It is important to note that this kind of electrostatic gating of a protonic (ionic) solution, unlike in nanofluidic devices, can occur for devices thicker than the Debye length ( k −1 ). From n 0 H+ , the maleic–chitosan ionic strength is ~1 mM, which results in k −1 ~ 10 nm. Even for the Figure 1a H + -FET, that is significantly thicker than the Debye length ( t ~8 k −1 ), V gs modulates I ds by changing the proton density of the channel. This is a unique property of having proton transparent contacts and reduces fabrication constraints. Device simulations We produce two-dimensional plots of the proton charge density n H+ at different V gs ( Fig. 4a–c ) by solving drift diffusion and Poisson equations in the context of a semiconductor device simulator, where the hole mobility is replaced by proton mobility. From these plots, it is clear that, for a negative V gs , the proton density is drastically increased at the polysaccharide–dielectric interface to form a highly conducting region. The thickness of this region (~10 nm) is in agreement with the estimated Debye length ( Fig. 4a ). Plots of current density show that the majority of I ds flows in the same area ( Supplementary Fig. S3 ). At the same time, a positive V gs considerably depletes the channel from protons reducing n H+ and consequently I ds ( Fig. 4c ). An analogous V gs effect on the charge density and current density distribution has been observed in thin-film organic transistors [34] . These transistors have geometry and electrostatics similar to our H + -FET. From these plots, it is also clear that in significantly thinner devices the expected charge modulation will be higher. Such devices may be fabricated with individual maleic–chitosan nanofibres and should offer a greatly improved on-off ratio. 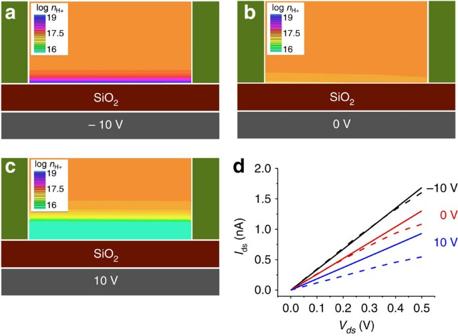Figure 4: Protonic Transistor Simulations. (a–c) two-dimensional plots of device nH+(log scale in cm−3) as a function ofVgs(Vds=0.3 V). (d) SimulatedIdsdata (lines) for smallVdscorresponding to device data shown inFigure 3a(only −10, 0, 10 Vgsshown for clarity). This data was generated usingn0H+=8.9×1017cm−3and a corresponding μsH+=5.5×10−3cm2V−1s−1, which is close to the one estimated from the device. The experimental data (dashed line) is shifted toIds=0 forVds=0 to compensate for hysteresis. Figure 4: Protonic Transistor Simulations. ( a–c ) two-dimensional plots of device n H+ (log scale in cm −3 ) as a function of V gs ( V ds =0.3 V). ( d ) Simulated I ds data (lines) for small V ds corresponding to device data shown in Figure 3a (only −10, 0, 10 V gs shown for clarity). This data was generated using n 0 H+ =8.9×10 17 cm −3 and a corresponding μ s H+ =5.5×10 −3 cm 2 V −1 s −1 , which is close to the one estimated from the device. The experimental data (dashed line) is shifted to I ds =0 for V ds =0 to compensate for hysteresis. Full size image We also estimate I ds as a function of V ds for different V gs ( Fig. 4d ). The simulations are in good agreement with the experimental data at low V ds , while the nonlinear dependence of I ds on V ds for higher V ds is not reproduced. We have assumed the contacts to be completely proton transparent. A small contact barrier (neglected in our model) may cause charge accumulation or depletion at the maleic–chitosan PdH x interface. This charge, in turn, may reduce the strength of the electric field at the contacts, thus effectively limiting the current. When the bias is reversed, the charge should be released and cause hysteresis in the I ds –V ds dependence. Hysteresis is indeed observed when V ds is ramped from 0 to 1 V and then back in the same measurement ( Supplementary Fig. S4 ). The causes for hysteresis and the non-linear behaviour of I ds for high V ds are still not fully understood and merit further investigation. These experiments demonstrate, for the first time, electrostatic gate modulation of source-drain current in a solid-state biopolymer based thin-film protonic (H + ) field-effect transistor. PdH x contacts allow for indiscriminate measurement of the protonic current. A voltage applied to the electrostatic gate controls the maleic–chitosan channel proton density and the channel conductivity. Current modulation occurs even for devices thicker than the Debye length. This allows for current control in highly concentrated electrolytes at any length scale. In the future, several nanostructured biological and organic materials can be measured in these devices. The demonstrated ability to control protonic currents in nanostructured biocompatible solid-state devices (bionanoprotonics) may open exciting opportunities for interfacing with living systems. These opportunities include biomedical applications where protonic currents are important such as the in-vivo study and stimulation of proton selective ion-channels. To this end, H + -FETs architectures with optimized performance in physiological solutions will be required. Maleic–chitosan nanofibres Maleic–chitosan nanofibres were prepared following previously published procedures [35] . The maleic–chitosan hydration level was determined with a thermogravimetric analyser (TA Instruments, model 2050). Two-terminal devices Cu contacts (1 cm 2 ×1 cm 2 ) coated with 50 nm e-beam evaporated (Balzers PLS 500) Pd (5 nm Cr adhesion layer) were used to sandwich 300 μm films for relative humidity (RH)-dependent measurements. Maleic–chitosan films were prepared from a 5 ml of 3.0 wt% maleic–chitosan aqueous solution after drying for 5 h. Chitin films were prepared from a 5 ml of 0.5 wt% chitin/HFIP solution after drying for 1 h. H + -FET Devices were fabricated on p-type Si (Addison Engineering, B, ρ =0.001 ohm cm −1 ) with thermally grown silicon oxide (100 nm). Photolithography and lift-off was used to define the contacts. Pd metal (50 nm) with a 5-nm Cr adhesion layer was deposited via e-beam evaporation (Balzers PLS 500). After dialysis and freeze drying, maleic–chitosan was prepared in a DI water solution. This procedure eliminates any salt and thus potential salt effects on the conductivity. To make a polysaccharide-based device, 2 μl polysaccharide solutions of concentration ranging from 0.02 mg ml −1 to 0.2 mg ml −1 were carefully drop cast on top of the patterned silicon wafer and blown under N 2 flow. Devices were mounted on a chip, and wire bonded. Electrical characterization Measurements were performed with a semiconductor parameter analyser (Agilent 4155C). An environmental chamber was used (5% H 2 or 100% N 2 ) with controlled RH monitored with a traceable hygrometer (Fisher Scientific, ±0.1% error). During pro-FET measurements at 75% RH and 5% H 2 , devices with no connections were monitored to have at most noise current. This was done to ensure that the measured device current was from the maleic–chitosan channel and not from water condensed on the top of the SiO 2 . Atomic force microscopy Atomic force microscopy (AFM) was employed to measure device dimensions. Tapping mode AFM was performed on a Veeco Multimode V with a Nanoscope IV controller using Veeco Probes Sb-doped Si cantilevers ( ρ =0.01–0.025 Ω-cm, k =40 N/m, ν ~300 kHz). Simulations Electrical properties of the structure were obtained by solving Poisson's equation together with the electron and hole (in this case, proton) continuity equations throughout a CAD tool (ATLAS, Silvaco). We defined a silicon (Si) based metal–oxide–semiconductor transistor with the same dimensions as the experiment. We used a 8.6-μm long, 3.5-μm wide, 82-nm channel with a rectangular cross-section sitting on the top of 100-nm SiO 2 gate dielectric ( ɛ sio2 =3.9). Pd ( Φ =5.1 eV) source and drain were modelled as ohmic protonic contacts (no barrier) to the material. We replaced the properties of silicon with those of the channel material. Maleic–chitosan ɛ mc =10, and n 0 =8.9×10 17 cm −3 from our estimate. Mobility was varied to fit the data. In addition, we assigned the mobility of electrons to a value that is orders of magnitude smaller than that of protons. This minimizes the role of electrons in the electrical response of the device. To calculate the gate capacitance, we first obtained the interface charge at different gate biases; whereas the two other contacts were kept at zero bias. The capacitance was then estimated by the simple equation of Δ Q/ Δ V, where Δ Q and Δ V represent the variations of the interface charge and gate, respectively. How to cite this article: Zhong, C. et al . A polysaccharide bioprotonic field-effect transistor. Nat. Commun. 2:476 doi: 10.1038/ncomms1489 (2011).